ARF triggers senescence inBrca2-deficient cells by altering the spectrum of p53 transcriptional targets ARF is a tumour suppressor activated by oncogenic stress, which stabilizes p53. Although p53 is a key component of the response to DNA damage, a similar function for ARF has not been ascribed. Here we show that primary mouse and human cells lacking the tumour suppressor BRCA2 accumulate DNA damage, which triggers checkpoint signalling and ARF activation. Furthermore, senescence induced by Brca2 deletion in primary mouse and human cells is reversed by the loss of ARF, a phenotype recapitulated in cells lacking RAD51. Surprisingly, ARF is not necessary for p53 accumulation per se but for altering the spectrum of genes activated by this transcription factor. Specifically, ARF enables p53 transcription of Dusp4 and Dusp7 , which encode a pair of phosphatases known to inactivate the MAP kinases ERK1/2. Our results ascribe a previously unanticipated function to the ARF tumour suppressor in genome integrity, controlled by replicative stress and ATM/ATR-dependent checkpoint responses. ARF tumour suppressor is encoded by the Ink4/Arf locus and is known to become activated upon oncogenic stress (reviewed in Gil and Peters [1] ). ARF inhibition allows cells under sustained oncogenic stress to proliferate; thus, its loss of function through deletion, mutation or epigenetic silencing is detected in various types of cancers. For example, ARF inactivation has been reported in 33% of colon carcinomas [2] , 25% of oligodendrogliomas [3] , 14% of breast tumours [4] , 26.5% of oral squamous carcinomas and 32–58% of gliomas [5] . Moreover, ARF exhibits tumour suppressor functions in mouse, as illustrated by the tumour susceptibility phenotype of ARF-deficient mice [6] , [7] . Oncogene signals activate ARF and generally elicit senescence-like cell cycle arrest. The best-characterized cellular function of ARF in this process is that of stabilizing p53 through the inhibition of MDM2, an E3 ubiquitin ligase that targets p53 for degradation [8] . Overexpressed ARF interacts directly with MDM2 and inhibits its ability to promote p53 degradation [9] , [10] , thereby enhancing the p53-dependent transcriptional response. It was thus expected that the tumour suppressor function of ARF would be p53-dependent. Indeed, ARF suppresses aberrant cell growth in response to oncogene activation, at least in part by inducing p53 (ref. 11 ). However, there is also evidence for a p53-indepenent function of ARF in tumour suppression [12] , as ARF can induce growth arrest in p53-deficient tumours. p53-independent functions of ARF can be explained by its multiple physical or functional interacting partners, which include nucleophosmin, E2F1, Myc, NF-κB, HIF-1α, ARF-BP1/Mule and ULF [1] , [12] . Oncogene overexpression has recently been identified as a source of genomic instability: through increased replication fork stalling and breakage, it promotes the elevated mutation rate characteristic of cancer cells [13] . DNA damage checkpoint kinases ATR and ATM are activated by oncogene signalling [14] and initiate the downstream events leading to growth arrest and/or cell death [15] . ATR is activated by single-stranded DNA (ssDNA), whereas ATM activation occurs primarily in response to double-strand breaks (DSBs). During oncogene overexpression, replicative lesions including replication fork stalling, premature or redundant origin firing and DNA hyper-replication lead to ATR activation [16] . This, in turn, triggers the phosphorylation of its downstream targets CHK1 and p53, leading ultimately to senescence and/or apoptosis. Similarly, ATM activation during oncogene overexpression by DSBs arising as secondary damage leads to p53/p21-dependent checkpoint responses and induction of cellular senescence [14] . Although both ARF- and ATM-dependent pathways are triggered by oncogene overexpression, whether they functionally interact with each other remains elusive. So far, lack of ARF induction in response to acute DNA damage caused by ionizing radiation has not excluded that ARF could be activated by other types of DNA damage [12] . Another important source of genomic instability found especially in hereditary cancers is directly linked to the presence of mutations in genes involved in homologous recombination (HR), a pathway involved in DNA DSB repair [13] . The tumour suppressor BRCA2 has a key role in HR repair reactions by promoting the assembly of RAD51, the central recombinase activity, at the sites of DNA breaks. Additionally, an essential function of the BRCA2/RAD51 complex distinct from its role in DSB repair is to protect stalled forks from nucleolytic degradation [17] , [18] . BRCA2 gene deficiency leads to accumulation of unrepaired DNA breaks, which undergo erroneous repair leading to chromosomal rearrangements, a hallmark of BRCA2-deficient cells and tumours [19] , [20] . In primary cells, this genomic instability leads to cell cycle arrest and embryonic lethality. In other words, the primary consequence of BRCA2 inactivation is less proliferation and is not the enhanced proliferation characteristic of tumour cells bearing BRCA2 gene mutations. Presumably, additional genetic alterations acquired during tumour development abrogate the mechanisms that would otherwise block tumour cell proliferation. p53 inactivation is the only mechanism known so far to promote tumour progression in BRCA2-deficient cells [21] . It is conceivable that mutations in factors other than p53 can similarly abrogate cell cycle arrest in HR-deficient cells. Here we demonstrate that ARF inactivation rescues senescence in BRCA2 -deficient mouse and human cells. ARF levels are elevated in response to Brca2 deletion and limit the proliferative capacity of these cells. ARF induction occurs post-transcriptionally and requires ATM/ATR-dependent signalling, as well as ssDNA formation through replicative stress. Importantly, we detect ARF accumulation in Brca2 -deficient mouse and human breast tumours, suggesting that ARF provides a tumorigenesis barrier in these cells. This protection mechanism is abrogated by the loss of p53. These results define a novel cellular function of the ARF tumour suppressor in the DNA damage response to genomic instability. Surprisingly, ARF induces senescence in response to inhibition of recombinational repair not merely by stabilizing p53 but by promoting transcription of a subset of its gene targets, including the dual specificity phosphatases dual specificity phosphatase 4 (DUSP)4 and DUSP7. Both enzymes act to inhibit the MAPK pathway through ERK1/2 dephosphorylation. We furthermore show that inhibiting the MAPK pathway through ERK1 abrogation is sufficient to suppress proliferation of BRCA2-deficient cells. This identifies for the first time the MAPK pathway as a key mechanism sustaining proliferation of HR-deficient cells. Brca2 deletion induces ARF expression in primary MEFs Persistent DNA breaks and illegitimate DSB repair caused by HR abrogation are hallmarks of Brca2 -deleted cells and tumours. To study the cellular responses to chronic DNA damage induced by Brca2 deletion and the impact of the p53 pathway in this response, we used primary MEFs established from mice carrying a conditional Brca2 allele [21] in a p53-proficient or -deficient background ( Brca2 F/− p53 +/+ and Brca2 F/− p53 −/− ). Transient expression of Cre recombinase from a self-inactivating retrovirus (Hit&Run; (ref. 22 )) resulted in efficient deletion of exon 11 and loss of Brca2 expression as monitored using western blotting ( Fig. 1a ). This was concomitant with robust phosphorylation of the DNA damage checkpoint kinase CHK2, indicative of an ATM-dependent DNA damage response. We also observed ARF accumulation at 4 and 6 days after adding selection to the Cre-treated samples, in contrast to uninfected control cells. The levels of ARF induction were similar in the presence or absence of p53, suggesting that it occurred independently of p53. 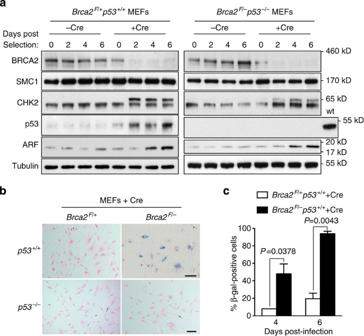Figure 1: The DNA damage response toBrca2conditional deletion induces ARF expression and senescence. (a) MEFs established fromBrca2F/−p53+/+andBrca2F/−p53−/−embryos were infected three times at 12-h intervals with retroviruses expressing self-deleting Cre recombinase (+Cre) or control pBabe empty vector (−Cre), then selected with puromycin for 48 h. Cell extracts were prepared at the indicated times after adding selection, and were analysed using western blotting. SMC1 and tubulin were used as loading controls. Wild-type (wt) MEFs were used as a control for p53 induction uponBrca2inactivation. (b) Cells treated with Cre as above were processed for SA-β-gal staining. Scale bar, 10 μm. (c) Quantification of the SA-β-gal staining shown in (b). Error bars represent s.d. of two independent experiments. The statistical significance of the β-gal response toBrca2deletion was evaluated using an unpaired two-tailedt-test. Figure 1: The DNA damage response to Brca2 conditional deletion induces ARF expression and senescence. ( a ) MEFs established from Brca2 F/− p53 +/+ and Brca2 F/− p53 −/− embryos were infected three times at 12-h intervals with retroviruses expressing self-deleting Cre recombinase (+Cre) or control pBabe empty vector (−Cre), then selected with puromycin for 48 h. Cell extracts were prepared at the indicated times after adding selection, and were analysed using western blotting. SMC1 and tubulin were used as loading controls. Wild-type (wt) MEFs were used as a control for p53 induction upon Brca2 inactivation. ( b ) Cells treated with Cre as above were processed for SA-β-gal staining. Scale bar, 10 μm. ( c ) Quantification of the SA-β-gal staining shown in ( b ). Error bars represent s.d. of two independent experiments. The statistical significance of the β-gal response to Brca2 deletion was evaluated using an unpaired two-tailed t -test. Full size image Brca2 deletion is known to lead to apoptosis and senescence in mice [21] because of activation of the p53 pathway. Consistent with this, we observed an increase in p53 levels in Brca2 F/− p53 +/+ MEFs upon Brca2 deletion, accompanied by the induction of senescence as determined with the senescence-associated β-galactosidase assay (SA-β-gal; Fig. 1b ). p53 −/− MEFs did not enter senescence following Brca2 gene inactivation, consistent with the idea that the loss of p53 function overcomes the proliferation defects in Brca2 -deficient cells [19] . Quantification of cells staining positive in the SA-β-gal assay showed an increase in the percentage of Brca2 −/− p53 +/+ cells entering senescence with time ( Fig. 1c ). As a control, Cre-treated cells carrying a wild-type Brca2 allele did not senesce under these experimental conditions, similarly to the p53 −/− MEFs. ATM mediates ARF induction in Brca2 -deficient cells Brca2 deletion triggered an ATM-dependent DNA damage response and ARF induction in MEFs ( Fig. 1a ). To investigate a possible link between the ATM response and elevated ARF levels, we suppressed ATM activity using the specific ATM inhibitor Ku55933 (ref. 23 ) in Cre-treated Brca2 F/− p53 +/+ MEFs. ATM inhibition reduced ATM and CHK2 phosphorylation in Brca2- deleted cells and also prevented ARF accumulation ( Fig. 2a ). These results suggested that activation of the ATM-dependent response in cells lacking Brca2 regulates ARF expression. 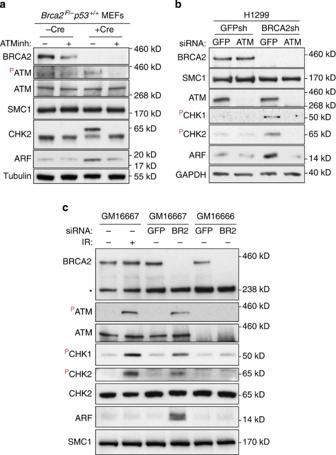Figure 2: ARF activation in BRCA2-deficient mouse and human cells is ATM-dependent. (a) MEFs established fromBrca2F/−p53+/+embryos were infected three times at 12-h intervals with retroviruses expressing self-deleting Cre recombinase (+Cre) or control pBabe empty vector (−Cre), in the presence or absence of ATM inhibitor Ku55933. SMC1 and tubulin were used as loading controls. (b) Human H1299 cells were infected with lentiviruses expressing control or BRCA2 shRNAs, followed by selection with puromycin for 48 h. Five days after infection, cells were transfected with control or ATM siRNAs. Cell extracts were prepared 6 days after infection and were analysed using western blotting. SMC1 and GAPDH were used as loading controls. (c) ATM-deficient GM16666 human cells and ATM-expressing GM16667 cells were transfected with control or BRCA2 siRNAs twice at 3 days interval. Extracts were prepared 6 days after the first transfection and immunoblotted as indicated. GM16667 cells used as control were irradiated (10 Gy) and extracts were prepared 2 h later. SMC1 was used as a loading control. *, nonspecific band. Figure 2: ARF activation in BRCA2-deficient mouse and human cells is ATM-dependent. ( a ) MEFs established from Brca2 F/− p53 +/+ embryos were infected three times at 12-h intervals with retroviruses expressing self-deleting Cre recombinase (+Cre) or control pBabe empty vector (−Cre), in the presence or absence of ATM inhibitor Ku55933. SMC1 and tubulin were used as loading controls. ( b ) Human H1299 cells were infected with lentiviruses expressing control or BRCA2 shRNAs, followed by selection with puromycin for 48 h. Five days after infection, cells were transfected with control or ATM siRNAs. Cell extracts were prepared 6 days after infection and were analysed using western blotting. SMC1 and GAPDH were used as loading controls. ( c ) ATM-deficient GM16666 human cells and ATM-expressing GM16667 cells were transfected with control or BRCA2 siRNAs twice at 3 days interval. Extracts were prepared 6 days after the first transfection and immunoblotted as indicated. GM16667 cells used as control were irradiated (10 Gy) and extracts were prepared 2 h later. SMC1 was used as a loading control. *, nonspecific band. Full size image To explore the dependence of ARF activation on ATM in human cells, we inhibited BRCA2 expression in H1299 cells using short hairpin RNA (shRNA) lentiviral constructs ( Fig. 2b ). We established two distinct shRNAs effective in depleting human BRCA2, which also induced ARF expression using western blotting ( Supplementary Fig. S1 ). BRCA2 depletion triggered an ATM-dependent response, illustrated by CHK2 phosphorylation ( Fig. 2b ), together with ARF upregulation, similarly to the Brca2 -deficient MEFs. As H1299 cells lack a functional p53 pathway [24] , they continued to proliferate in spite of HR abrogation. Importantly, inhibition of ATM expression using short interfering RNA (siRNA) in the BRCA2-depleted cells silenced the DNA damage response and abolished ARF accumulation. We employed ATM -deficient ataxia telangiectasia human fibroblasts transduced with empty vector (GM16666 cells) or wild-type ATM (GM16667 cells) to further validate the dependency of ARF induction on ATM. We found that complete BRCA2 abrogation using siRNA in these cells required two rounds of siRNA delivery at 3-day intervals ( Fig. 2c ). Upon BRCA2 depletion, ATM-proficient fibroblasts mounted a DNA damage response, as seen by the phosphorylation of ATM and its substrates (ATM, CHK1 and CHK2), comparable to that induced by exposure to ionizing radiation. ARF accumulation was not detected in cells exposed to 10 Gy of ionizing radiation, supporting the notion that ARF is not part of the fast, acute DNA damage response, as previously reported [25] . Together, these results indicate that ATM promotes ARF induction in response to BRCA2 deficiency in mouse and human cells. ssDNA formation leads to ARF induction in HR-deficient cells We next explored the dependency of ARF induction on downstream effectors of the ATM signalling cascade. ATM activation leads to MRE11-RAD50-NBS1 (MRN)-dependent DSB resection with the formation of ssDNA [26] . The nucleolytic activity of MRE11 is critical for end-processing reactions [27] . To investigate whether MRE11 is required for ARF induction in BRCA2-deficient cells, we inhibited BRCA2 expression in H1299 human cells using shRNA lentiviral constructs and MRE11, using mirin. BRCA2 protects stalled replication forks from MRE11-dependent nucleolytic degradation [17] ; thus, we predicted that BRCA2 deficiency would cause ssDNA accumulation. To detect ssDNA in cells lacking BRCA2, we used flow cytometry of BrdU-incorporating cells, in which BrdU antibody staining was detected under non-denaturing conditions [28] . BRCA2 depletion in human cells triggered a robust ssDNA signal ( Fig. 3a ), which was effectively suppressed by treatment with the MRE11 nuclease inhibitor mirin [29] . MRE11-dependent ssDNA formation is the signal for ATR activation. Consistent with this, mirin treatment abolished CHK1 phosphorylation, the signature of ATR activation, in BRCA2-depleted cells, whereas ATM-dependent CHK2 phosphorylation remained unaffected ( Fig. 3b ). Importantly, ARF induction was abolished when cells lacking BRCA2 were cultured in the presence of mirin, indicating the dependence of ARF accumulation on MRE11 activity. 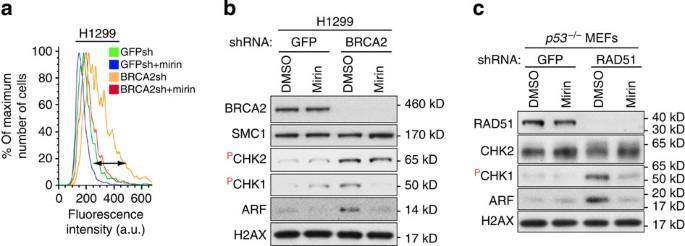Figure 3: MRE11-dependent ssDNA formation triggers ARF induction in BRCA2- and RAD51-deficient cells. (a) Human H1299 cells were infected with lentiviruses expressing control or BRCA2 shRNAs, followed by selection with puromycin for 48 h, in the presence or absence of MRE11 inhibitor mirin. Single-stranded DNA in these cells was quantified using FACS analysis of BrdU immunofluorescence detected under non-denaturing conditions. (b) Cell extracts from cells treated as inawere prepared 6 days after infection and analysed using western blotting. SMC1 and H2AX were used as loading controls. (c) MEFs established fromp53−/−embryos were treated with GFP control or RAD51 shRNAs followed by selection with puromycin for 48 h, in the presence or absence of MRE11 inhibitor mirin. Extracts were prepared from cells collected 6 days after infection and immunoblotted as indicated. Histone H2AX was used as a loading control. Figure 3: MRE11-dependent ssDNA formation triggers ARF induction in BRCA2- and RAD51-deficient cells. ( a ) Human H1299 cells were infected with lentiviruses expressing control or BRCA2 shRNAs, followed by selection with puromycin for 48 h, in the presence or absence of MRE11 inhibitor mirin. Single-stranded DNA in these cells was quantified using FACS analysis of BrdU immunofluorescence detected under non-denaturing conditions. ( b ) Cell extracts from cells treated as in a were prepared 6 days after infection and analysed using western blotting. SMC1 and H2AX were used as loading controls. ( c ) MEFs established from p53 −/− embryos were treated with GFP control or RAD51 shRNAs followed by selection with puromycin for 48 h, in the presence or absence of MRE11 inhibitor mirin. Extracts were prepared from cells collected 6 days after infection and immunoblotted as indicated. Histone H2AX was used as a loading control. Full size image BRCA2 acts as the loader of RAD51, a key enzyme for recombinational DNA repair, at break sites or stalled replication forks [30] . To examine the validity of this response in mouse cells lacking RAD51, we inhibited RAD51 expression using shRNA in p53 –/– MEFs. These cells are known to proliferate in spite of DNA damage accumulation [31] . Both ATM-dependent checkpoint activation and elevated ARF levels triggered by BRCA2 deficiency were recapitulated in cells lacking RAD51 ( Fig. 3c ). Similarly to Brca2- deleted MEFs, ARF accumulation and CHK1 phosphorylation were reduced to control levels upon treatment with mirin. Thus, ARF induction requires MRE11 activity in human and mouse cells lacking core components of the HR reaction. ARF induction by HR deficiency or oncogenes is ATR-dependent MRE11-dependent ssDNA accumulation in BRCA2-deficient cells required ATM, but not ATR, activation ( Supplementary Fig. S2a,b ). Moreover, MRE11-dependent ssDNA formation triggered ATR signalling, as indicated by CHK1 phosphorylation ( Fig. 3b,c ). To investigate the contribution of the ATR kinase to ARF induction in BRCA2-depleted human cells, we downregulated ATR using an shRNA lentiviral construct ( Fig. 4a ) or inactivated it using a chemical inhibitor [32] ( Supplementary Fig. S3 ). Both treatments abolished ARF induction triggered by BRCA2 depletion. Similarly, ATR chemical inhibition led to reduction in ARF levels in RAD51-depleted MEFs ( Fig. 4b ). As a control, CHK1 phosphorylation, the signature of ATR activation, was effectively diminished by this treatment. Similarly to Brca2- deleted MEFs, ARF accumulation was attenuated by treatment with the ATM inhibitor Ku55933 in mouse cells lacking RAD51 ( Fig. 4b ). In addition, inducing replication stress with hydroxyurea (HU) treatment led to significant ssDNA accumulation ( Supplementary Fig. S4a ). Strikingly, HU-treated cells showed elevated ARF expression, in addition to an ATM/ATR-dependent DNA damage response indicated by CHK2 and CHK1 phosphorylation ( Supplementary Fig. S4b ). Both the increase in ARF levels and the phosphorylation of the two checkpoint kinases were abrogated by treatment with ATM or ATR inhibitors. 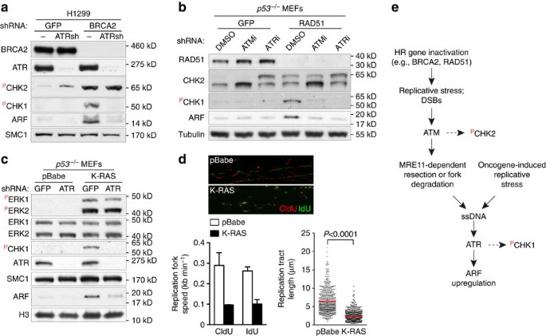Figure 4: ATR induces ARF expression in response to HR deficiency or oncogenic stress. (a) Human H1299 cells were infected with lentiviruses expressing indicated shRNAs, followed by selection with puromycin for 48 h. Cell extracts were prepared 6 days after infection and were analysed using western blotting. SMC1 was used as a loading control. (b) MEFs established fromp53−/−embryos were infected three times with control or RAD51 shRNAs, in the presence or absence of ATM or ATR chemical inhibitors (ATMi, ATRi). Extracts prepared from cells collected 6 days after the first infection were immunoblotted as indicated. Tubulin was used as a loading control. (c) MEFs established fromp53−/−embryos were infected with control or K-RAS-expressing retroviruses, in the presence of control or ATR shRNAs. Extracts prepared from cells collected 6 days after the first infection were immunoblotted as indicated. ERK, SMC1 and H3 were used as loading controls. (d) Quantification of replication fork speed and tract length using single DNA fibre analysis in cells treated as inc. Error bars represent s.d. of two independent experiments. The statistical significance of the observed reduction in replication tract length induced by K-RAS expression was evaluated using an unpaired two-tailedt-test. Representative images of ongoing replication forks identified with CldU and IdU staining are also shown. (e) Schematic diagram of the DNA damage response to replicative stress, leading to ARF accumulation. Figure 4: ATR induces ARF expression in response to HR deficiency or oncogenic stress. ( a ) Human H1299 cells were infected with lentiviruses expressing indicated shRNAs, followed by selection with puromycin for 48 h. Cell extracts were prepared 6 days after infection and were analysed using western blotting. SMC1 was used as a loading control. ( b ) MEFs established from p53 −/− embryos were infected three times with control or RAD51 shRNAs, in the presence or absence of ATM or ATR chemical inhibitors (ATMi, ATRi). Extracts prepared from cells collected 6 days after the first infection were immunoblotted as indicated. Tubulin was used as a loading control. ( c ) MEFs established from p53 −/− embryos were infected with control or K-RAS-expressing retroviruses, in the presence of control or ATR shRNAs. Extracts prepared from cells collected 6 days after the first infection were immunoblotted as indicated. ERK, SMC1 and H3 were used as loading controls. ( d ) Quantification of replication fork speed and tract length using single DNA fibre analysis in cells treated as in c . Error bars represent s.d. of two independent experiments. The statistical significance of the observed reduction in replication tract length induced by K-RAS expression was evaluated using an unpaired two-tailed t -test. Representative images of ongoing replication forks identified with CldU and IdU staining are also shown. ( e ) Schematic diagram of the DNA damage response to replicative stress, leading to ARF accumulation. Full size image ARF expression is induced by oncogene signalling, also known to trigger replicative stress and accumulation of DNA damage in a less acute manner than IR exposure [15] . We therefore explored the possibility that oncogene-mediated ARF induction is triggered by the DNA damage inflicted by oncogene overexpression. To investigate this, we expressed K-RAS, an oncogenic form of RAS, in p53 −/− MEFs. ERK1/2 phosphorylation, a signature of K-RAS signalling activation [33] , was detected in these cells 5 days after infection ( Fig. 4c ). Although ARF accumulation occurred in response to oncogene expression, p53 deficiency enabled these cells to proliferate. We monitored replication in these cells using DNA fibre analysis ( Fig. 4d ). Cells expressing oncogenic RAS showed a marked replication fork slow-down and a striking shortening of the replication tract compared with the control cells. These results suggested a correlation between oncogene-induced replication stress and ARF upregulation. Consistent with the notion that oncogenic RAS triggers replicative stress and DNA damage signalling [34] , we also detected CHK1 phosphorylation, suggestive of ATR activation ( Fig. 4c ). Surprisingly, shRNA-mediated ATR inhibition in K-RAS-expressing p53 −/− MEFs not only abrogated CHK1 phosphorylation but also ARF induction. This indicated that oncogene-driven induction of ARF is ATR-dependent and occurs in response to DNA damage. We attempted to inhibit ATR expression in p53 +/+ cells. This, however, led to proliferative arrest and cell death precluding further investigation. Taken together, these results demonstrate that ARF upregulation in response to the loss of recombinational repair or to oncogene activation is the consequence of DNA damage accumulation and ATM/ATR-dependent signalling ( Fig. 4e ). ARF induction in response to oncogene activation can be regulated either transcriptionally or at a post-translational level [1] . To investigate whether ARF was transcriptionally induced upon BRCA2 abrogation, ARF mRNA levels were monitored using quantitative PCR. Interestingly, ARF mRNA levels did not change significantly upon BRCA2 depletion in human H1299 cells ( Supplementary Fig. S5a ). In addition, E2F1, a well-characterized ARF transcription factor and ATM phosphorylation substrate [35] , was not required for ARF accumulation in BRCA2-deficient GM16667 human fibroblasts ( Supplementary Fig. S5b ). Taken together, these results suggest that ARF induction in response to HR deficiency is not regulated at the transcriptional level. To address mechanistically the observed transcription-independent ARF accumulation, we determined the half-life of ARF protein in H1299 cells lacking BRCA2. Although ARF is unstable in cultured cells [36] , its half-life was markedly increased in response to BRCA2 shRNA-mediated depletion ( Supplementary Fig. S6a, b ). Importantly, ARF ubiquitylation detectable upon proteasome inhibition with MG132 ( Supplementary Fig. S6c ) was reduced upon BRCA2 inhibition. This suggested that the ubiquitylation reactions, which target ARF for degradation under normal physiological conditions, are either inhibited or reversed in response to HR abrogation, leading to protein stabilization. ARF inactivation rescues senescence in Brca 2-deficient cells Elevated levels of ARF expression activate a transcriptional network, leading to proliferation arrest and senescence via downregulation of MDM2 (ref. 1 ). Brca2 deletion in MEFs triggered both an increase in ARF levels and senescence onset, suggesting the possibility that ARF induction is required for the senescence response in these cells. To address this, we depleted ARF in Brca2 F/− p53 +/+ MEFs using shRNA. Consistent with the above results, Cre-mediated deletion of Brca2 led to an increase in ARF levels as determined using western blotting ( Fig. 5a ), which was efficiently suppressed by treatment with ARF shRNA. As a control, ARF shRNA did not affect p16 protein levels, the second transcript encoded by the Ink4b-ARF-Ink4a locus ( Supplementary Fig. S7a ). Brca2 deletion led to a robust induction of senescence in the Cre-treated cells ( Figs 1b,c and 5b ), which was almost completely abrogated by two independent shRNAs against mouse ARF ( Fig. 5b ). Both shRNAs were effective in lowering ARF mRNA levels when transduced into MEFs, whereas Cre-mediated Brca2 deletion alone did not alter ARF transcription patterns ( Supplementary Fig. S8a ). Inhibiting ARF expression also restored proliferation in Brca2 -deleted MEFs ( Supplementary Fig. S9a ). This suggested that ARF activation is required for p53-mediated senescence in cells lacking BRCA2. 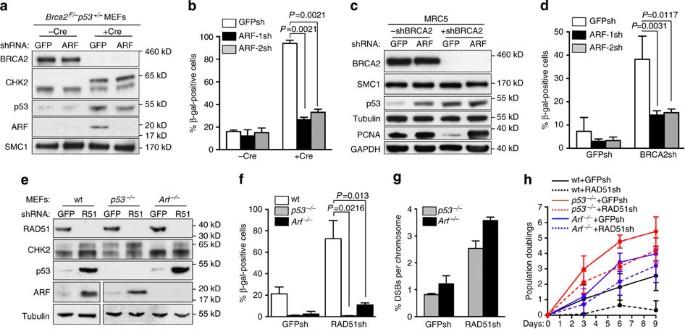Figure 5: ARF inhibition rescues senescence and proliferation arrest induced by BRCA2 or RAD51 inactivation in mouse and human cells. (a) Early-passage MEFs established fromBrca2F/−p53+/+embryos were infected three times at 12-h intervals with retroviruses expressing self-deleting Cre recombinase (+Cre) or control pBabe empty vector (−Cre), together with retroviruses expressing ARF or GFP control shRNA, followed by selection with puromycin for 48 h. Cell extracts were prepared 6 days after the first infection and were analysed using western blotting. SMC1 was used as a loading control. (b) Quantification of the SA-β-gal staining of cells treated as ina. Error bars represent s.d. of two independent experiments. The statistical significance of the β-gal response to concomitantBrca2deletion and ARF depletion was evaluated using an unpaired two-tailedt-test. ARF-1sh and ARF-2sh are two independent shRNAs against mouse ARF. (c) Human MRC5 cells were infected with lentiviruses expressing indicated shRNAs, followed by selection with puromycin for 48 h. Cell extracts were prepared 6 days after infection and were analysed using western blotting. SMC1, GAPDH and tubulin were used as loading controls. (d) Quantification of the SA-β-gal staining of cells treated as inc. Error bars represent s.d. of two independent experiments. The statistical significance of the β-gal response to concomitant BRCA2 and ARF depletion was evaluated using an unpaired two-tailedt-test. (e) Early-passage MEFs established from wild-type,p53−/−orArf −/−embryos were treated with GFP control or RAD51 shRNAs. Extracts were prepared from cells collected 6 days after infection and immunoblotted as indicated. Tubulin was used as a loading control. (f) Quantification of the SA-β-gal staining of cells treated as in (e). Error bars represent s.d. of two independent experiments. The statistical significance of the β-gal response to RAD51 depletion in the three types of MEFs was evaluated using an unpaired two-tailedt-test. ARF-1sh and ARF-2sh are two independent shRNAs against human ARF. (g) Quantification of the DSBs frequency in metaphase spreads from cells treated as ine. (h) Cell proliferation assays for cells treated as ine. Error bars represent s.d. of three independent experiments. Figure 5: ARF inhibition rescues senescence and proliferation arrest induced by BRCA2 or RAD51 inactivation in mouse and human cells. ( a ) Early-passage MEFs established from Brca2 F/− p53 +/+ embryos were infected three times at 12-h intervals with retroviruses expressing self-deleting Cre recombinase (+Cre) or control pBabe empty vector (−Cre), together with retroviruses expressing ARF or GFP control shRNA, followed by selection with puromycin for 48 h. Cell extracts were prepared 6 days after the first infection and were analysed using western blotting. SMC1 was used as a loading control. ( b ) Quantification of the SA-β-gal staining of cells treated as in a . Error bars represent s.d. of two independent experiments. The statistical significance of the β-gal response to concomitant Brca2 deletion and ARF depletion was evaluated using an unpaired two-tailed t -test. ARF-1sh and ARF-2sh are two independent shRNAs against mouse ARF. ( c ) Human MRC5 cells were infected with lentiviruses expressing indicated shRNAs, followed by selection with puromycin for 48 h. Cell extracts were prepared 6 days after infection and were analysed using western blotting. SMC1, GAPDH and tubulin were used as loading controls. ( d ) Quantification of the SA-β-gal staining of cells treated as in c . Error bars represent s.d. of two independent experiments. The statistical significance of the β-gal response to concomitant BRCA2 and ARF depletion was evaluated using an unpaired two-tailed t -test. ( e ) Early-passage MEFs established from wild-type, p53 −/− or Arf −/− embryos were treated with GFP control or RAD51 shRNAs. Extracts were prepared from cells collected 6 days after infection and immunoblotted as indicated. Tubulin was used as a loading control. ( f ) Quantification of the SA-β-gal staining of cells treated as in ( e ). Error bars represent s.d. of two independent experiments. The statistical significance of the β-gal response to RAD51 depletion in the three types of MEFs was evaluated using an unpaired two-tailed t -test. ARF-1sh and ARF-2sh are two independent shRNAs against human ARF. ( g ) Quantification of the DSBs frequency in metaphase spreads from cells treated as in e . ( h ) Cell proliferation assays for cells treated as in e . Error bars represent s.d. of three independent experiments. Full size image The role of ARF in cell proliferation is differentially regulated in mouse and human cells [1] , [24] . Thus, we next investigated whether ARF is required for the senescence induced by BRCA2 inactivation in human cells. Transduction of MRC5 human primary fibroblasts with lentiviruses encoding BRCA2 shRNA ( Fig. 5c ) inhibited BRCA2 expression and resulted in 38% of the cells entering senescence. Diminished PCNA expression was used as a marker for senescence, efficiently reversed by concomitant ARF inhibition ( Fig. 5c ). ARF expression in these cells was not detectable using western blotting; instead, using quantitative PCR (QPCR) we established that the two independent hairpins targeting human ARF in MRC5 cells did not affect p16 levels ( Supplementary Fig. S7b ), that they effectively downregulated ARF mRNA levels ( Supplementary Fig. S8b ) and rescued senescence induced by BRCA2 depletion ( Fig. 5d , Supplementary Fig. S9b ). To gain a better understanding of ARF regulation in response to HR deficiency, we depleted RAD51 from wild-type Arf −/− and p53 −/− MEFs using shRNA. We found that the DNA repair phenotypes characteristic of BRCA2 deficiency are recapitulated in cells lacking RAD51. Specifically, we detected activation of the ATM pathway illustrated by CHK2 phosphorylation in the three types of MEFs ( Fig. 5e ). Moreover, similarly to BRCA2 inactivation, RAD51 depletion induced p53 and ARF expression and increased senescence in wild-type MEFs. Over the course of 5 days following shRNA infection, this resulted in 73% of the cells in the wild-type population entering senescence ( Fig. 5f ). Importantly, the senescence response was significantly diminished when RAD51 was depleted in either Arf −/− or p53 −/− MEFs (11 and 1% senescent cells, respectively). Although p53 accumulation was detectable in Arf −/− MEFs upon inhibition of RAD51 ( Fig. 5e ), this increase in p53 expression was not sufficient to elicit a senescence response, which indicates that ARF is essential for the cell cycle arrest induced by HR abrogation. We observed the accumulation of unrepaired chromosome breaks in the three types of MEFs treated with RAD51 shRNA ( Fig. 5g ). In wild-type MEFs, this led to proliferative arrest ( Fig. 5h ), which substantially limited the number of metaphase chromosomes available for DSB quantification. In contrast, Arf −/− and p53 −/− MEFs continued to proliferate following RAD51 depletion ( Fig. 5h ), in spite of DSB accumulation. This demonstrates that ARF inactivation silenced the DNA damage checkpoint, which underlies the mechanism of ARF impact on genome integrity. ARF is upregulated in Brca2 -deficient mammary tumours To determine whether the DNA damage response and ARF upregulation observed in Brca2 -deleted MEFs are also features of Brca2 -deficient tumours, we used immunohistochemistry to examine sections from tumours induced in the mammary epithelium of p53 F/F and p53 F/F Brca2 F/F mice by Cre-mediated deletion [21] ( Fig. 6a ). Both single p53 -deleted ( n =10) and doubly p53 - and Brca2 -deleted ( n =9) tumours showed a high frequency of γH2AX staining (~50% of cells stained positive for this marker), indicative of DNA damage response activation ( Fig. 6b ). In contrast, ARF staining was seen in only 14% of cells in control p53-negative tumours but in 25% of cells in Brca2, p53- deficient tumours. This was a modest, but statistically significant, increase in cells that show ARF induction associated with loss of the Brca2 gene. We also examined the frequency of γH2AX and ARF staining in tumour microarrays from human sporadic breast tumours ( n =65) and compared it to breast tumours from carriers of BRCA2 mutations ( n =40; Fig. 6c ). Sporadic tumours showed γH2AX staining in 77% of cells on average ( Fig. 6d ), similarly to tumours from BRCA2 -deficient individuals in which γH2AX staining was found in 83% of cells on average. Strikingly, 49% of the cells examined in BRCA2 -deficient tumours stained positive for ARF, compared with only 27% of cells in sporadic tumours. These results indicate that the DNA damage response, as well as the ARF pathway, are activated in BRCA2 -deficient tumours. Analysis of p21 expression in a subset of the human breast tumours showed that increased ARF expression correlated with the loss of p53 function ( Supplementary Fig. S10 ), similarly to the mouse mammary tumours. This suggests that the increase in ARF levels, which would normally limit proliferation, may be counteracted by p53 inactivation during progression of BRCA2 -deficient cells to tumorigenesis. 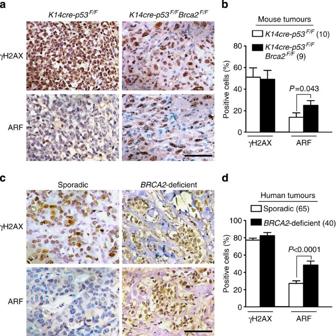Figure 6: Elevated ARF expression inBrca2-deficient mouse and human breast tumours. (a) Sections fromK14cre-p53F/FBrca2F/Fand controlK14cre-p53F/Fmouse mammary tumours were stained with antibodies against γH2AX and ARF. Nuclei were counterstained with hematoxylin. Scale bar, 45 μm. (b) Quantification of the percentage of cells scored positive for each antibody marker. The number of tumours examined is shown in brackets. Bars represent s.d. The statistical significance of increased ARF staining inBrca2-deficient tumours was evaluated using an unpaired two-tailedt-test. (c) Sections from sporadic andBRCA2-mutated human breast tumours were stained with antibodies against γH2AX and ARF. Nuclei were counterstained with hematoxylin. Scale bar, 40 μm. (d) Quantification of the percentage of cells scored positive for each antibody marker. The number of tumours examined is shown in brackets. Bars represent s.d. The statistical significance of increased ARF staining inBRCA2-mutated tumours was evaluated using an unpaired two-tailedt-test. Figure 6: Elevated ARF expression in Brca2 -deficient mouse and human breast tumours. ( a ) Sections from K14cre-p53 F/F Brca2 F/F and control K14cre-p53 F/F mouse mammary tumours were stained with antibodies against γH2AX and ARF. Nuclei were counterstained with hematoxylin. Scale bar, 45 μm. ( b ) Quantification of the percentage of cells scored positive for each antibody marker. The number of tumours examined is shown in brackets. Bars represent s.d. The statistical significance of increased ARF staining in Brca2- deficient tumours was evaluated using an unpaired two-tailed t -test. ( c ) Sections from sporadic and BRCA2 -mutated human breast tumours were stained with antibodies against γH2AX and ARF. Nuclei were counterstained with hematoxylin. Scale bar, 40 μm. ( d ) Quantification of the percentage of cells scored positive for each antibody marker. The number of tumours examined is shown in brackets. Bars represent s.d. The statistical significance of increased ARF staining in BRCA2- mutated tumours was evaluated using an unpaired two-tailed t -test. Full size image Nevertheless, it is clear that some BRCA2-deficient human cancer cell lines and tumours carry ARF deletions. Whether ARF loss could reverse the proliferative block and drive tumorigenesis in cells lacking BRCA2 was an unanswered question. We therefore analysed ARF and p53 mutation frequencies in a collection of 742 human cancer cell lines (Sanger Institute). Our results ( Supplementary Table S1 ) indicate a lower frequency of ARF loss in BRCA2 -deleted compared with BRCA2 wild-type cells, in contrast to p53 inactivation, which occurs at similar levels in both types of cells. ARF mediates p53-dependent transcription of Dusp4 and Dusp7 Our data indicate that ARF is not required to stabilize p53 in response to DNA damage accumulation triggered by HR abrogation, as Arf −/− MEFs showed an increase in p53 levels upon RAD51 depletion ( Fig. 5e ). Similarly, p53 induction was observed in MEFs and MRC5 cells in which BRCA2 and ARF were simultaneously inactivated ( Fig. 5a,c ). Nevertheless, p53 induction in RAD51-depleted Arf −/− MEFs was not sufficient to trigger senescence in these cells ( Fig. 5f ), suggesting that ARF modulates the ability of p53 to efficiently inhibit cell proliferation. Post-translational modifications are known to regulate the cellular functions of p53. Among these, Ser18 phosphorylation (Ser15 in human) is required for p53 activation after DNA damage [6] . As anticipated, we detected p53 Ser18 phosphorylation in wild-type cells in response to shRNA-mediated RAD51 depletion ( Supplementary Fig. S11 ). In contrast, Arf −/− MEFs lacked p53 Ser18 phosphorylation and showed a compensatory increase in total p53 levels. Post-translational modifications of p53 alter its binding affinity to specific DNA sequences within promoters and impact on transcription of its target genes [37] . As p53 Ser18 phosphorylation is not detectable in RAD51-depleted Arf −/− MEFs, we anticipated that the expression profile of these cells, in particular that of p53 transcriptional targets, is different from that of RAD51-depleted wild-type MEFs. Using mRNA microarray analysis and expression profiling, we identified genes upregulated in wild-type primary MEFs treated with RAD51 shRNA, whose expression was not induced in similarly treated Arf −/− primary MEFs ( Fig. 7a ). Clustering analysis of p53 transcriptional targets with increased expression in RAD51-depleted cells revealed the following three groups: genes requiring functional ARF for their expression, genes transcribed in an ARF-independent manner and genes those are upregulated in both ARF-proficient and ARF-deficient cells ( Fig. 7b ). Among the genes in the last group, we found Cdkn1a(p21), encoding the p21 inhibitor of cyclin-dependent kinases and well-characterized effector of the p53 role in promoting senescence [38] . The subset of p53 targets requiring ARF for their transcription was specifically upregulated in response to RAD51 inhibition in wild-type but not in Arf −/− MEFs. Among these genes, two encoded the DUSP family members DUSP4 and DUSP7, which act as ERK phosphatases and negative regulators of the MAPK kinase pathway in mammalian cells [39] . To validate the results of microarray analyses, we monitored the mRNA levels of Cdkn1a(p21), Dusp4 and Dusp7 transcripts using quantitative RT–PCR ( Fig. 7c ). Cdkn1a(p21) mRNA was upregulated in response to RAD51 inhibition in both wild-type and Arf −/− MEFs, whereas Dusp4 and Dusp7 transcription was only induced in wild-type MEFs. Thus, ARF is required for p53-mediated transcription of Dusp4 and Dusp7 in RAD51-depleted cells, unlike Cdkn1a(p21) whose expression increased independently of ARF. 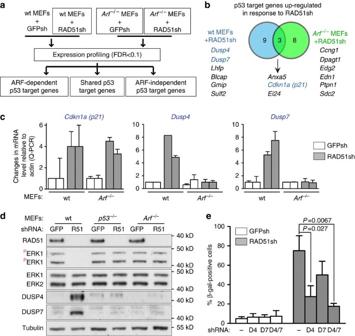Figure 7: ARF implements the checkpoint through p53-dependent transcriptional upregulation of DUSP4/7 and ERK dephosphorylation. (a) Schematic overview of mRNA expression profiling. Early-passage MEFs established from wild-type orArf−/−embryos were treated with RAD51 or GFP control shRNA. Total RNA was extracted from cells collected 4 days after infection and hybridized to mRNA expression arrays. p53 transcriptional targets were grouped as shown. (b) p53 target genes upregulated in response to RAD51 shRNA-mediated inhibition specifically in wild-type orArf−/−MEFs, as well genes shared between the two are indicated. Gene lists were obtained from the analysis of microarray data from three independent experiments. (c) The mRNA levels ofCdkn1a,Dusp4andDusp7genes were determined using quantitative PCR in cells treated as ina. (d) Early-passage MEFs established from wild-type,p53−/−orArf−/−embryos were treated with GFP control or RAD51 shRNAs. Extracts were prepared from cells collected 6 days after infection and immunoblotted as indicated. Tubulin was used as a loading control. (e) Quantification of the SA-β-gal staining of early-passage MEFs established from wild-type embryos and treated with indicated shRNAs. Error bars represent s.d. of two independent experiments. The statistical significance of the β-gal response to DUSP4 or DUSP4/7 co-depletion in RAD51 shRNA-treated wild-type MEFs was evaluated using an unpaired two-tailedt-test. D4, DUSP4; D7, DUSP7. Figure 7: ARF implements the checkpoint through p53-dependent transcriptional upregulation of DUSP4/7 and ERK dephosphorylation. ( a ) Schematic overview of mRNA expression profiling. Early-passage MEFs established from wild-type or Arf −/− embryos were treated with RAD51 or GFP control shRNA. Total RNA was extracted from cells collected 4 days after infection and hybridized to mRNA expression arrays. p53 transcriptional targets were grouped as shown. ( b ) p53 target genes upregulated in response to RAD51 shRNA-mediated inhibition specifically in wild-type or Arf −/− MEFs, as well genes shared between the two are indicated. Gene lists were obtained from the analysis of microarray data from three independent experiments. ( c ) The mRNA levels of Cdkn1a , Dusp4 and Dusp7 genes were determined using quantitative PCR in cells treated as in a . ( d ) Early-passage MEFs established from wild-type, p53 −/− or Arf −/− embryos were treated with GFP control or RAD51 shRNAs. Extracts were prepared from cells collected 6 days after infection and immunoblotted as indicated. Tubulin was used as a loading control. ( e ) Quantification of the SA-β-gal staining of early-passage MEFs established from wild-type embryos and treated with indicated shRNAs. Error bars represent s.d. of two independent experiments. The statistical significance of the β-gal response to DUSP4 or DUSP4/7 co-depletion in RAD51 shRNA-treated wild-type MEFs was evaluated using an unpaired two-tailed t -test. D4, DUSP4; D7, DUSP7. Full size image We next addressed the roles of DUSP4 and DUSP7 in the senescence response to HR inactivation. Both DUSP4 and DUSP7 protein levels were induced in wild-type but not in Arf −/− or p53 −/− MEFs upon RAD51 depletion ( Fig. 7d ), which was consistent with the observed upregulation of their mRNA levels ( Fig. 7c ). DUSP4 and DUSP7 inductions were also detected after Brca2 Cre-mediated deletion in primary wild-type MEFs ( Supplementary Fig. S12a ). Elevated DUSP4 and DUSP7 levels were associated with abrogation of P-ERK1/2 phosphorylation, consistent with their established role in dephosphorylating ERK1/2 kinases [40] . Loss of ERK1/2 phosphorylation inhibits the MAPK pathway and promotes cell cycle arrest. Importantly, shRNA-mediated inhibition of DUSP4 ( Supplementary Fig. S12b ) reversed the senescence phenotype of RAD51-depleted MEFs ( Fig. 7e ) and partially restored proliferation ( Supplementary Fig. S9c ). Additional inactivation of DUSP7 ( Supplementary Fig. S12c ) further enhanced the effects on senescence and cell proliferation. DUSP4 shRNA inhibition partially restored ERK1/2 phosphorylation ( Supplementary Fig. S13 ). Loss of DUSP7 expression alone did not significantly decrease senescence of HR-deficient cells ( Fig. 7e ) but restored ERK1/2 phosphorylation to levels similar to DUSP4 inhibition ( Supplementary Fig. S13 ). Thus, DUSP4-specific targets may be very important to bypass senescence in response to HR abrogation in primary MEFs. ERK1 is required for proliferation of BRCA2-deficient cells DUSP4 and DUSP7 have high specificity for ERK1/2 in in vitro phosphatase assays [39] . We thus examined the impact of ERK1/2 inhibition on the proliferation of BRCA2-deficient cells. Human CAPAN-1 cells are derived from a pancreatic epithelial tumour and carry only one BRCA2 allele, which encodes a truncated form of the protein localized to the cytoplasm [41] . Treatment of CAPAN-1 cells with shRNAs against ERK1 and ERK2 effectively abolished expression of each of the two proteins ( Fig. 8a ). Whereas ERK2 depletion had only a modest effect on CAPAN-1 proliferation compared with control cells, ERK1 inhibition suppressed cell growth and essentially killed the BRCA2-deficient cells ( Fig. 8b ). The same effect was recapitulated using two additional independent shRNAs against ERK1 ( Supplementary Fig. S14a,b ). Importantly, treatment of CAPAN-1 cells with ERK1 shRNA triggered apoptosis, as indicated by the increase in cleaved PARP levels using western blotting and by elevated sub-G1 fraction determined in FACS analyses of the DNA content ( Supplementary Fig. S14c,d ). We next attempted to recapitulate the effects of ERK1 shRNA-mediated inhibition using chemical inhibitors. Instead of ERK inhibitors, which proved to be cytotoxic in clinical trials, we used inhibitors of the upstream kinases MEK1/2. BRCA2-defective hamster cells [42] were highly susceptible to growth defects induced by the MEK inhibitor, in contrast to isogenic cells in which BRCA2 expression was ectopically restored ( Fig. 8c ). 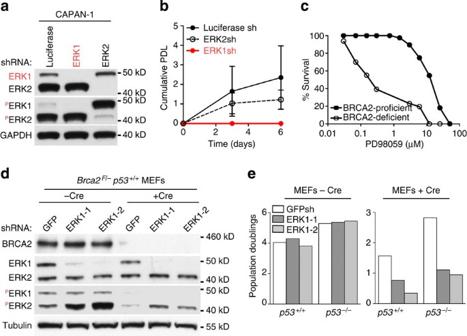Figure 8: shRNA-mediated ERK1 depletion inhibits proliferation in BRCA2-deficient human and mouse cells. (a) Human CAPAN-1 cells were transduced twice at a 24-h interval with lentiviruses expressing ERK1, ERK2 or luciferase control shRNA, followed by selection with puromycin for 72 h. Cell extracts were prepared 24 h later and were analysed using western blotting. GAPDH was used as a loading control. (b) Cell proliferation assays for cells treated as ina. Error bars represent s.d. of three independent experiments. PDL, population doublings. (c) Susceptibility of BRCA2-deficient (V-C8) and proficient (V-C8+BRCA2) hamster cells to MEK1/2 inhibitor PD98059. Percentage survival was measured using a clonogenic survival assay70. (d) MEFs established fromBrca2F/−p53+/+embryos were infected three times at 12-h intervals with retroviruses expressing self-deleting Cre recombinase (+Cre) or control pBabe empty vector (−Cre). The same MEFs were transduced twice with lentiviruses expressing two independent shRNAs against mouse ERK1 (ERK1-1, ERK1-2) or GFP control shRNA, followed by selection with puromycin for 48 h. Cell extracts prepared 48 h later were immunoblotted as indicated. Tubulin was used as a loading control. (e) Population doublings of cells treated as indwere determined 6 days after the removal of selection. Figure 8: shRNA-mediated ERK1 depletion inhibits proliferation in BRCA2-deficient human and mouse cells. ( a ) Human CAPAN-1 cells were transduced twice at a 24-h interval with lentiviruses expressing ERK1, ERK2 or luciferase control shRNA, followed by selection with puromycin for 72 h. Cell extracts were prepared 24 h later and were analysed using western blotting. GAPDH was used as a loading control. ( b ) Cell proliferation assays for cells treated as in a . Error bars represent s.d. of three independent experiments. PDL, population doublings. ( c ) Susceptibility of BRCA2-deficient (V-C8) and proficient (V-C8+BRCA2) hamster cells to MEK1/2 inhibitor PD98059. Percentage survival was measured using a clonogenic survival assay [70] . ( d ) MEFs established from Brca2 F/− p53 +/+ embryos were infected three times at 12-h intervals with retroviruses expressing self-deleting Cre recombinase (+Cre) or control pBabe empty vector (−Cre). The same MEFs were transduced twice with lentiviruses expressing two independent shRNAs against mouse ERK1 (ERK1-1, ERK1-2) or GFP control shRNA, followed by selection with puromycin for 48 h. Cell extracts prepared 48 h later were immunoblotted as indicated. Tubulin was used as a loading control. ( e ) Population doublings of cells treated as in d were determined 6 days after the removal of selection. Full size image We further tested the validity of this result in mouse cells. Inhibiting ERK1 expression with two independent shRNAs ( Fig. 8d ) significantly reduced the proliferation of MEFs carrying a Cre-mediated Brca2 -deletion, irrespectively of their p53 status ( Fig. 8e ). A similar inhibition of cell proliferation was observed in BRCA2-depleted U2OS cells treated with ERK1 shRNA ( Supplementary Fig. S15a,b ). Inhibition of ERK2 in these cells had no effect on cell cycle progression. This result has important clinical implications, as loss of p53 is a common occurrence in human BRCA2 -defective tumours. BRCA2-proficient cells were not markedly affected by ERK inactivation, suggesting that the BRCA2 deficiency specifically sensitizes cells to the antiproliferative effect of ERK1 inhibition. Several lines of evidence link acute oncogenic signalling with ARF transcriptional activation. The same oncogenes that induce ARF also trigger replication stress and DNA damage, leading to ATM/ATR activation and CHK-dependent signalling to senescence [14] , [43] . Although the contribution of p53 to the response to DNA damage is well characterized, previous studies failed to establish a clear role for ARF in this process [1] . Here we report that ARF expression is upregulated in mouse and human cells in response to replicative stress and chronic accumulation of unrepaired DNA damage triggered by HR abrogation or exposure to a 5-day regime of oncogene signalling. Importantly, our MEF experiments have all been performed in low-oxygen conditions, which enabled us to exclude spontaneous increase in ARF levels [44] and accumulation of oxygen-radical-induced DNA damage [45] associated with normal oxygen culture conditions. Our results demonstrate that ARF is a key component of the ATM/ATR-dependent response to DNA damage. Mutations in the human tumour suppressor BRCA2 are linked to the onset of a large number of hereditary breast and ovarian cancers. The major cellular role of BRCA2 is to load a key DNA repair enzyme, RAD51, on DNA ends at sites of DNA breaks induced by genotoxic treatments. BRCA2 also binds and protects stalled replication forks from nucleolytic degradation under physiological cell cycle conditions [17] , [18] . In addition, we have recently demonstrated that BRCA2 has a second role in maintaining genome stability, to facilitate telomere replication, as well as to prevent telomeres from uncapping and thus becoming an intrinsic source of genomic instability [31] . Both these functions account for the high levels of spontaneous chromosomal aberrations seen in BRCA2-defective cells (reviewed by Venkitaraman [20] ). The original paradigm for ARF cellular functions is based on induction and stabilization of p53. Although the role of p53 in the response to DNA damage is well characterized, previous results failed to establish a clear link between the DNA damage response and ARF activation [1] . DNA damage responses are diminished in Arf -deficient MEFs, which do not undergo cell cycle arrest in response to ionizing radiation [25] ; however, this has been interpreted as attenuated p53 function. A possible reason for the lack of evidence for ARF activation by DNA damage is the fact that damage responses are usually assessed after high-dose irradiation or genotoxic treatments [25] , [44] . The acute response relies on MDM2 inhibition to allow immediate stabilization of p53 and to prevent further proliferation of cells carrying damaged DNA [46] . Here we demonstrate that ARF is not part of this fast, acute DNA damage response; however, it is activated by replication stress and chronic DNA damage following abrogation of repair pathways essential for genome integrity. ARF induction is a rather slow process, which is probably one of the reasons for being overlooked in studies using high-dose DNA damage, which activates acute, rapid cellular responses. We demonstrate that in cells lacking BRCA2 or RAD51, replicative stress triggered ARF accumulation in an ATM/ATR-dependent manner. We monitored several steps of the DNA-damage-signalling cascade in these cells and found that ATM activity, MRE11-mediated resection and ATR function are required for ARF activation. Importantly, we demonstrate that replication stress caused by oncogene overexpression similarly elicited ARF induction in an ssDNA- and an ATR-dependent manner. This indicates that the DNA damage response is a potent trigger of ARF activation. Contrary to previous models [35] , ARF accumulation was not regulated at the transcriptional level. The slow kinetics of ARF induction in response to chronic DNA damage could be explained by the observed stabilization of the protein through reduced ubiquitylation and degradation. Interestingly, ULF1, an E3 ubiquitin ligase previously shown to regulate ARF turnover in response to oncogenic stress [36] , was not required for the response to HR abrogation. As ULF1 action is modulated by nucleophosmin, also a target of the ATM-dependent response to DNA damage [47] , we anticipate that this cofactor is also not required in this context. This may suggest that yet undefined regulatory mechanisms govern ARF stability in cells lacking recombinational repair. As BRCA2 mediates repair processes critical for genome integrity, its loss leads to lethality during embryonic development or severe proliferation defects in normal, noncancerous cells in culture. Consistent with this, we demonstrate here that conditionally deleted Brca2 MEFs stop dividing in culture and enter senescence triggered by ARF and p53 induction. Paradoxically, BRCA2-defective tumour cells are characterized by a high proliferative capacity, suggesting that additional mutations are acquired during tumour development, which abrogate vital mechanisms that limit malignant progression. p53 inactivation was the only genetic alteration known so far to allow BRCA2-deficient tumour cells to expand. However, conditional deletion of BRCA2 in p53 −/− genetic background only partially rescues embryos viability [19] , suggesting that factors additional to p53 are required to maintain the cell cycle arrest. In this study, we identified ARF inhibition as a new mechanism to rescue senescence in BRCA2-defective cells. Our results demonstrate that Arf -null MEFs and human cells fail to senesce in response to chronic DNA damage induced by deletion of the key HR repair factors (that is, BRCA2 and RAD51). These cells accumulate unrepaired DNA breaks but fail to enter cell cycle arrest proliferation, indicting a checkpoint defect. This identifies an unanticipated key role for ARF in the chronic DNA damage response leading to senescence in cells lacking recombinational repair. Surprisingly, abrogation of senescence occurs in spite of p53 induction in Arf −/− MEFs or in ARF shRNA-treated human MRC5 cells, suggesting that ARF is required in addition to p53 to promote senescence under chronic damage conditions. Our results are consistent with the observation that p53 expression alone is not a sufficient tumour suppressor of lymphomas in Arf -null mice [48] . Conversely, p53 −/− MEFs fail to senesce in response to chronic DNA damage, in spite of elevated ARF levels. This observation is of particular relevance to our clinical data showing that ARF is upregulated specifically in Brca2 -deficient mouse and human breast tumours. All mammary tumours examined show high levels of γH2AX staining, indicative of DSB induction and ATM-dependent checkpoint activation, a common feature of precancerous lesions [43] . In a Brca2 -defective background, unrepaired DSBs persist and can be detected in the fully developed breast tumours analysed here. Thus, if Brca2 inactivation is the initiating event in these tumours, it is expected that the antitumorigenic response, illustrated by ATM activation and ARF induction in our panel of tumours, will block proliferation. However, ARF upregulation is a slow response and, thus, it is likely that the severe genomic instability induced by the loss of BRCA2 could lead to p53 inactivation before ARF can accumulate and initiate the cellular responses leading to senescence. p53 abrogation could restore the proliferative potential of these cells and initiate tumorigenesis. Our results therefore provide a possible explanation for the common loss of p53 function observed in Brca -deficient breast tumours [21] , [49] , [50] : p53-deficient cells might be selected as possessing efficient means to counteract the tumorigenic barrier imposed by ARF activation. Probably the most surprising of our results is that ARF is required to alter the spectrum of genes that are activated by p53. Unexpectedly, HR deficiency does not limit cellular proliferation in Arf -null cells, in spite of p53 induction. This implies that ARF is not merely required to stabilize p53 in order to sustain the senescence response to Brca2 deletion. Instead, it acts to change the expression of a set of p53 target genes, which are required to implement senescence. Post-translational p53 modifications determine its DNA-binding affinity to specific sequences within promoters and the transcriptional activation of its targets [37] . We demonstrate that ARF is required for p53 Ser18 phosphorylation in response to DNA damage. Indeed, Arf −/− MEFs lacked p53 Ser18 phosphorylation triggered by RAD51 inactivation. This was surprising because ATM/ATR signalling was activated in these MEFs. Direct protein–protein interactions between ATM/ATR and ARF have been previously reported [51] . It is therefore possible that ARF acts to facilitate substrate recognition or as a cofactor in ATM/ATR-dependent p53 phosphorylation reactions. This, in turn, may mediate the ability of p53 to activate a specific subset of gene targets. Indeed, ARF is required for expression of p53 transcriptional targets Dusp4 and Dusp7 , encoding two phosphatases with largely unknown physiological functions [39] . At the molecular level, DUSP4 and DUSP7 inhibit cell proliferation through dephosphorylation of ERK1/2 kinases, which abrogates the MAPK pathway. This could predict a causative link between the elevated levels of DUSP4 and DUSP7 and the senescence phenotype in RAD51-depleted cells. Abnormalities in the MAPK signalling pathways have been implicated in a wide range of human malignancies. The classical ERK pathway has long been known to be associated with lifespan extension of cancer cells and is upregulated in ~30% of human tumours [39] . Consistent with this, we find that inhibiting DUSP4, alone or in combination with DUSP7, can reverse the proliferation arrest in RAD51-depleted cells, most likely by restoring ERK1/2 phosphorylation and MAPK signalling. Expression and activity of DUSPs are differentially regulated in cells and tissues and determine the amplitude of the MAPK response leading to distinct physiological outcomes [40] . Notably, low levels of DUSP4 expression were recently reported to be associated with resistance to adjuvant chemotherapies in breast cancer patients [52] , which is in line with our data showing increased proliferation of HR-deficient cells upon inhibition of DUSP4 expression ( Fig. 7e ). Although the precise function of DUSP4 in the healthy tissue remains unclear, this observation may nevertheless be suggestive of specific DUSP4 regulation in tissues, which are prone to Brca2 loss-induced tumorigenesis. Our data suggest a model in which loss of recombinational repair triggers ARF expression. This, in turn, induces p53 transcriptional targets DUSP4 and DUSP7 ( Fig. 9 ), two phosphatases acting to promote senescence through ERK1/2 dephosphorylation and inhibition of the MAPK pathway. Importantly, we demonstrate that inhibition of ERK1, but not ERK2, is sufficient to inhibit proliferation of BRCA2 -deficient cells. ERK1 deletion accelerates the rate of cell death triggered by the loss of Brca2 and is therefore synthetically lethal with Brca2 deletion. ERK1 inhibitors may identify tractable targets from a pharmacological point of view and may function similarly to PARP inhibitors [42] , [53] to target and eliminate specifically BRCA2-defective tumour cells. We demonstrate that ERK1 inhibition eliminates BRCA2-defective cells regardless of their p53 status. This observation has clinical relevance, as it suggests that suppressing ERK1 may be effective in targeting broad spectrum of Brca2 -deficient cells and tumours, including those lacking p53 (refs 21 , 49 , 50 ). 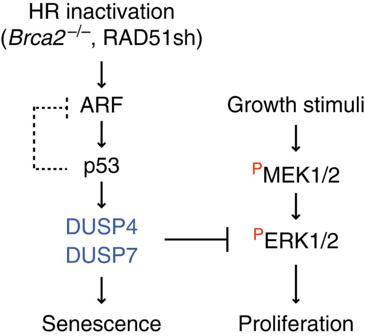Figure 9: Schematic diagram of the senescence response in HR-deficient primary cells. ARF accumulation stimulates p53-dependent transcription of DUSP4/7 phosphatases. A negative feedback regulatory loop through p53 on ARF expression also exists. DUSP4/7 acts to inhibit the MAPK survival pathway through ERK1/2 dephosphorylation. Figure 9: Schematic diagram of the senescence response in HR-deficient primary cells. ARF accumulation stimulates p53-dependent transcription of DUSP4/7 phosphatases. A negative feedback regulatory loop through p53 on ARF expression also exists. DUSP4/7 acts to inhibit the MAPK survival pathway through ERK1/2 dephosphorylation. Full size image It is surprising in this context to note that ERK2, a MAPK family member closely related to ERK1, does not compensate for the loss of ERK1 function in these cells. Although activatory ERK2 phosphorylation is detected in BRCA2-lacking cells, it is possible that ERK2 downstream phosphorylation targets are not sufficiently potent to sustain survival. This target specificity further highlights the well-characterized functional dichotomy of the ERK1 and ERK2 kinases [54] , initially suggested by the observation that lethality triggered by ERK2 deletion in mice is not compensated by ERK1. In summary, abrogating the MAPK pathway either by DUSP activation or ERK1 inhibition triggers cell cycle arrest in cells lacking BRCA2 expression. This establishes MAPK signalling as a key mechanism for the survival of HR-deficient cells. These considerations have important clinical implications, as modalities of MAPK pathway inhibition could lead to growth arrest or rapid elimination of HR-defective cells and tumours. The antitumorigenic potential of MEK kinase inhibitors, enzymes known to phosphorylate and activate ERK1/2, is currently under clinical evaluation. One prediction from our results is that patients with known HR defects (for example, carriers of BRCA1, BRCA2, RAD51C or RAD51D mutations) may benefit most from these therapies. Cell culture and treatments Cervical cancer cell line HeLa OHIO, pancreatic cancer cell line CAPAN-1 (both from CR-UK Cell Services), lung cancer cell line H1299, primary human fibroblasts MRC5 (both from American Type Culture Collection), BRCA2-mutated hamster cells transduced with empty vector or BRCA2 (V-C8 and V-C8+BRCA2, respectively [42] ; gifts from Dr. T. Helleday) and ataxia telangiectasia-mutated fibroblasts transduced with empty vector or ATM (GM16666 and GM16667, respectively; Coriell Institute Repository) were cultivated in monolayers in DMEM medium (Sigma Aldrich) supplemented with 10% foetal bovine serum (Life Technologies), penicillin and streptomycin (Sigma Aldrich). Primary wild-type or p53 −/− MEFs [55] were isolated from day 13.5 embryos as previously described [56] . Briefly, individual 13.5 dpc embryos were washed in phosphate-buffered saline (PBS) and placed in individual 10-cm dishes for dissection. Following removal of the red organs, embryos were trypsinized on ice to generate a homogenous cell suspension. MEFs established from individual embryos were further cultivated in DMEM medium (Sigma Aldrich) supplemented with 10% foetal bovine serum (Life Technologies), penicillin and streptomycin (Sigma Aldrich) in a low-oxygen (3%) incubator. Brca2 F/+ and Brca2 −/+ mice [21] in p53 +/+ or p53 −/− background were crossed to obtain E13.5 Brca2 F/− p53 +/+ or Brca2 F/− p53 −/− fetuses from which MEFs were established. Arf −/− MEFs were a gift from M. Serrano (CNIO, Madrid). ATM inhibitor Ku55933 (ref. 23 ; a gift from Graeme Smith), ATR inhibitor [32] (Vertex Pharmaceuticals) or dimethylsulphoxide solvent were added to the cells at 10 and 2 μM final concentrations, respectively. For mitotic arrest, cells were treated with 0.1 μg ml −1 colcemid overnight. HU (Sigma Aldrich) was added to a final concentration of 2 mM. Mirin (Sigma Aldrich) was added to the cells to a final concentration of 25 μM. Hamster V-C8 and V-C8+BRCA2 cells were grown in the presence of the indicated concentrations of MEK1/2 inhibitor PD98059 (Cell Signalling) for the entire duration of the clonogenic survival assay. siRNAs H1299, GM16666 and GM16667 were transfected using Oligofectamine (Life Technologies) or Dharmafect 1 (Dharmacon Research). Briefly, 2 × 10 6 cells were transfected with 40 nM siRNA per plate by reverse transfection in 10-cm plates. For transfections with BRCA2 siRNA, cells were replated 3 days after the first transfection in the 10-cm plates (2 × 10 6 cells per plate) and transfected again as above. Three days after the last siRNA transfection, cells were collected by trypsinization and processed for immunoblotting. siRNA duplexes were 21-base pairs long with 2-base deoxynucleotide overhang. The sequence of BRCA2 siRNA was 5′-UCAGCUGGCUUCAACUCCAUU-3′ and ATM siRNA was 5′-AAGGCUAUUCAGUGUGCGAGA-3′ (Qiagen). A GFP siRNA with the sequence 5′-GCUGACCCUGAAGUUCAUCUU-3′ was used as a control. Retroviral transduction of MEFs and human cells Retroviral transduction of primary MEFs was performed as described [57] . Briefly, HEK293T packaging cells were grown to 70% confluency and transfected with pCL-Eco helper vector together with either pBabe plus retroviral vector encoding ‘Hit-and-run’ Cre recombinase [22] or pBabe alone using a standard calcium phosphate protocol. Where indicated, a construct of mutant K-RasV12 cloned into pBabe (9052, Addgene) was similarly transfected into HEK293T packaging cells. For shRNA transfection, retroviral constructs in pRetroSuper encoding control GFP [58] , human p14 ARF -1 (5′-GAACAUGGUGCGCAGGUUC), human p14 ARF -2 (5′-GAACATGGTGCGCAGGTTC-3′), mouse p19 ARF -1 (ref. 59 ), mouse p19 ARF -2 (5′-GTTCGTGCGATCCCGGAGA-3′; a gift from Rene Bernards, NKI, Amsterdam), mouse RAD51 (ref. 31 ), mouse ATR [60] , mouse DUSP4 (5′-GTCTCTTCAGACTGTCCCAAT-3′) and mouse DUSP7 (5′-CCATAACCTGTTCCCGATCAA-3′) shRNAs were transfected along with pCL-Eco helper vector. The cell supernatant was collected 24 h after transfection. Recipient MEFs, U2OS or MRC5 cells were plated 24 h before their first infection with the retroviral supernatants. Additional infections were performed after 24 and 32 h. Twenty-four hours after the last infection, cells were washed and incubated in fresh medium containing 2–3 μg ml −1 puromycin for 2 days. Exponentially growing cells were either collected and processed for immunoblotting, RT–qPCR and SA-β-gal staining or were arrested in mitosis by addition of colcemid and processed for metaphase spreads preparation as described below. Lentiviral transduction of MEFs and human cells Lentiviral transduction was performed as previously described [61] . Briefly, HEK293T packaging cells were grown to 70% confluency and transfected with gag-pol, Res-Rev and VSV-G packaging vectors together with pLKO.1 constructs encoding the following shRNAs: control GFP [58] , control luciferase [62] , human ATR (5′-CCGGAUACUUACAGAUGUAAA-3′), human BRCA2-1 (5′-UCAGCUGGCUUCAACUCCAUU-3′), human BRCA2-2 (5′-ACAACAAUUACGAACCAAAC-3′), mouse ERK1-1 (5′-CAUGCUUAAUUCCAAGGGCUA-3′), mouse ERK1-2 (5′-CAUUAACAUGAAGGCCCGAAA-3′), human ERK1-1 (5′-GCCAUGAGAGAUGUCUACA-3′; ref. 63 ), human ERK1-2 (5′-UCCCUGUCAAAGCUGUCACUU-3′), human ERK1-3 (5′-CGUGCUCCACCGAGAUCUAAA-3′), human ERK2 (5′-GAGGAUUGAAGUAGAACAG-3′; ref. 63 ). The cell supernatant was collected 24 h after transfection. Recipient cells were plated and infected twice at 12-h intervals with the lentiviral supernatants. Twenty-four hours after the last infection, cells were washed thoroughly and incubated in fresh medium containing 2–3 μg ml −1 puromycin for 3–5 days. Exponentially growing cells were collected and processed as described for the retroviral transduction. SA-β-galactosidase staining The SA-β-gal staining was adapted from previously described protocols [64] . Briefly, cells were washed in PBS, fixed with 2% formaldehyde, 0.2% glutaraldehyde for 10–15 min at room temperature and washed again in PBS. Cells were stained by incubation with freshly prepared staining solution (1 mg ml −1 X-Gal, 5 mM potassium ferrocyanide, 5 mM potassium ferricyanide, 150 mM NaCl, 2 mM MgCl 2 , 40 mM citric acid, pH 6.0) at 37 °C with atmospheric CO 2 levels. Staining became evident in 2–4 h and was stopped after 12–16 h. Cells were stained with Nuclear Fast Red solution (Sigma Aldrich) before examination using light microscopy. Proliferation assay MEFs were seeded at 1 × 10 4 cells per well in 24-well plates. Cell number was determined at 3, 6 and 9 days after plating by incubating the cells with media containing 10 μg ml −1 of resazurin for 2 h. Fluorescence was measured at 590 nm using a plate reader (EnVision, Perkin Elmer). Preparation of metaphase spreads Mitotic cells were collected by mitotic shake-off and swollen in hypotonic buffer (0.03 M sodium citrate, pH 7.5) at 37 °C for 25 min. Cells were fixed in a freshly prepared 3:1 mix of methanol:glacial acetic acid, dropped on slides pre-soaked in 45% acetic acid and left to dry overnight. Fluorescence in situ hybridization (FISH) staining was performed with a telomeric FISH probe as previously described [58] . The frequency of DNA breaks was calculated as the total number of chromatid and chromosome breaks per number of chromosomes analysed. DNA fibre analysis Single-molecule DNA fibre analysis was performed as previously described [65] . Briefly, cells were pulse-labelled with 25 μM CldU for 1 h, washed three times with PBS and pulse-labeled with 250 μM IdU for 1 h. Labelled cells were collected and resuspended in cold PBS. The cell suspension was mixed with lysis buffer (0.5% SDS, 50 mM EDTA, 200 mM Tris-Cl, pH 7.4) and spotted on a microscope slide, which was tilted in a 15° angle to allow spreading of the genomic DNA into single-molecule DNA fibres by gravity. DNA spreads were air-dried, fixed-denatured in 2.5 M HCl and used for CldU and IdU detection using immunofluorescence. The length of red- or green-labelled streaks was measured using the ImageJ software (National Institutes of Health) and arbitrary length values were converted into micrometres using the scale bars created using the microscope. The rate for nascent replication tract degradation was estimated using the conversion of 2.59 kb μm −1 . Immunohistochemical analysis of tissue samples Formalin-fixed tissue samples were processed for immunohistochemical staining as previously described [14] . Briefly, 5-mm thick paraffin sections were mounted on poly- L -lysine-coated slides, dewaxed, rehydrated and incubated for 15 min with 3% hydrogen peroxide to quench the endogenous peroxidase activity. Antigen retrieval was carried out using 10 mM citric acid buffer pH 6.0 in a steamer for 15 min. The second-generation polymer method (UltraVision LP, LabVision, Anti-Sel-Greece) was used for signal detection according to the manufacturer’s instructions. For colour development, we used 3,3'-diaminobenzidine tetrahydrochloride (LabVision) and hematoxylin as a counterstain. The following mouse monoclonal antibodies were used for immunohistochemical analysis: anti-γH2AX (pSer139) (Millipore, dilution 1:100), anti-p19 ARF (Santa Cruz Biotechnology, dilution 1:100), anti-p14 ARF (Abcam, dilution 1:100), anti-p21 (Leica Microsystems, dilution 1:20). Immunoblotting Cells were collected by trypsinization, washed twice with PBS and resuspended in SDS–PAGE loading buffer and sonicated. Equal amounts of protein (50–100 μg) were analysed using gel electrophoresis followed by western blotting. NuPAGE-Novex 10% Bis-Tris gels or Tris-Acetate 3–8% (Life Technologies) were run according to the manufacturer’s instructions. ssDNA assay Detection of ssDNA under non-denaturing conditions was performed as in Bunting et al. [28] Cells were pulsed with BrdU (Sigma Aldrich) for 48 h, collected by trypsinization, fixed in ice-cold 70% ethanol overnight at −20 °C and stained under non-denaturing conditions with anti-BrdU antibody (Becton Dickson). At least 10,000 cells in the S/G2 phase of the cell cycle were analysed using flow cytometry (Becton Dickson). mRNA microarray expression profiling Total RNA was extracted with Trizol (Life Technologies) and hybridized to mRNA expression arrays (HumanWG-6 BeadChip; Illumina) in accordance with the manufacturer’s instructions ( http://microarrays.nki.nl ). Data were normalized with quantile normalization (GEO submission: NCBI tracking system #16887520) and further analysed with the EXPANDER package. Background correction was carried out by variance-stabilizing transformation available in the Bioconductor’s lumi package [66] . Differentially expressed genes were obtained by fitting linear models with the limma package [67] . To account for multiple hypothesis testing, the estimated significance level ( P -value) was adjusted using Benjamini and Hochberg false discovery rate correction. Those genes with false discovery rate <0.1 were selected as being differentially expressed. Quantitative RT–PCR To determine ARF mRNA levels in H1299 and MRC5 cells following shRNA-mediated depletion of ARF, real-time RT–PCR using the Power SYBR Green Cells-to-Ct kit (Ambion) was performed 3 days post selection. The primer set 1 used to amplify ARF mRNA in MRC5 cells was: 5′-CCGCCGCGAGTGAGGGTTTT-3′ and 5′-GCCCATCATCATGACCTGGTCTTCT-3′ and primer set 2: 5′-TTCACATCCCGCGGCTCACG-3′ and 5′TCATGACCTGGTCTTCTAGGAAGCG-3′. Real-time RT–PCR was similarly used to determine endogenous mRNA levels of Cdkn1a, Dusp4 and Dusp7 after RAD51 shRNA treatment in MEFs. The primer set for Cdkn1a was 5′-CGCTGCGTGACAAGAGAATA-3′ and 5′-CCTCCCCTCTGGGAATCTAA-3′, for Dusp4 : 5′-TCTACTCGGCTGTCATCGT-3′ and 5′-TCTCATAGCCACCTTTAAGCA-3′ and for Dusp7 : 5′-AATACATCCTCAACGTCACAC-3′ and 5′-GGGCTTCATCAATGAAGCTG-3′. Primers for human 18S (5′-AGTCCCTGCCCTTTGTACACA-3′ and 5′-GATCCGAGGGCCTCACTAAAC-3′) and mouse β−actin (5′-GCTCTGGCTCCTAGCACCAT-3′ and 5′-CCACCGATCCACACAGAGTAC-3′) were used as endogenous controls. Antibodies The following antibodies were used in immunoblotting: rabbit polyclonal antisera raised against ATM (Sigma Aldrich), H2AX (Calbiochem), SMC1 (Bethyl Laboratories), CHK1 (Cell Signalling Technology), phosphorylated CHK1 (Ser 345, Cell Signalling Technology), phosphorylated CHK2 (Thr 68, Cell Signalling Technology), RAD51 (Santa Cruz Biotechnology), p14 (Abcam), p16 (Santa Cruz Biotechnology), p53 (Santa Cruz Biotechnology), ERK (Cell Signalling Technology), full-length PARP (9542, Cell Signalling Technology), cleaved PARP Asp214 (9541, Cell Signalling Technology), phospho-p53 Ser15 (Cell Signalling Technology), E2F1 (Santa Cruz Biotechnology), DUSP4 (Santa Cruz Biotechnology), DUSP7 (Abcam) and human histone H3 (a gift from A. Verreault); mouse monoclonal antibodies raised against BRCA2 (OP95, Calbiochem), CHK2/Cds1 (Upstate), P-ERK (Cell Signalling Technology), phosphorylated ATM (Cell Signalling Technology), GAPDH (Novus Biologicals), PCNA (Santa Cruz Biotechnology) and α-tubulin [68] (Cancer Research UK Monoclonal Antibody Service); rat monoclonal antibody against p19 (Novus); goat polyclonal antibody raised against ATR (Santa Cruz Biotechnology) and sheep polyclonal antibody raised against BRCA2 (ref. 69 ). How to cite this article: Carlos, A. R. et al. ARF triggers senescence in Brca2 -deficient cells by altering the spectrum of p53 transcriptional targets. Nat. Commun. 4:2697 doi: 10.1038/ncomms3697 (2013).